Electric field-induced chemical locomotion of conducting objects Externally triggered motion of small objects has potential in applications ranging from micromachines, to drug delivery, and self-assembly of superstructures. Here we present a new concept for the controlled propulsion of conducting objects with sizes ranging from centimetres to hundreds of micrometres. It is based on their polarization, induced by an electric field, which triggers spatially separated oxidation and reduction reactions involving asymmetric gas bubble formation. This in turn leads to a directional motion of the objects. Depending on the implied redox chemistry and the device design, the speed can be controlled and the motion can be switched from linear to rotational. This type of chemical locomotion is an alternative to existing approaches based on other principles. The design and study of objects that can move in a controlled way and perform tasks at small scales has attracted huge interest across many areas of science ranging from biology to physics. Intensive studies have been performed in order to imitate biomotors [1] by developing molecular motors [2] , [3] and also synthetic micro- and nanomotors [4] , [5] . Several original strategies have been explored to induce motion of artificial 'swimmers', the most developed ones being the chemically powered motors. Various mechanisms, including bubble propulsion, diffusiophoresis, self-electrophoresis and bioelectrochemical propulsion have been proposed and studied in this context [6] , [7] , [8] , [9] . So far, different exciting applications such as writing of microstructures [10] , DNA detection [11] , isolation of cancer cells [12] or drug delivery [13] have been explored, and several groups are concentrating their efforts on the design [14] , [15] , [16] , the synthesis [17] , [18] and on the motional control of the swimmers to push forward this interdisciplinary field of research. To avoid the use of chemical fuel, alternative mechanisms are also investigated. Magnetic field-induced motion can be very efficient at the microscale, as has been shown by Ghosh et al . [19] and Dreyfus et al . [20] Electric field-driven motion is also a very promising area. Electrokinetic phenomena are known to occur on particles when exposed to an electric field and can be used to move the objects [21] . In uniform DC fields, charged particles migrate towards the electrode of opposite charge. In uniform AC fields, diodes can be propelled in a controlled way [22] , [23] . Non-uniform AC fields can also be exploited because of dielectrophoretic forces [24] , inducing motion at the micro- and nanoscale, with applications in areas such as sorting of nanotubes [25] , cell separation [26] and colloidal crystal assembly [27] . The key concept for the propulsion of particles is to break the symmetry of the system, and thus a majority of previously described techniques require the use of intrinsically asymmetric swimmers in order to generate controlled motion. This point is important because asymmetric structures are difficult to obtain from a synthetic point of view and most of the approaches, which are used to break the symmetry require interfaces [28] . One alternative approach is through the use of bipolar electrochemistry, whose principle relies on the fact that when a conducting particle is placed in an electric field, a maximum polarization voltage Δ V occurs between the two sides of the particle oriented towards the electrodes. This voltage is proportional to the electric field E and the characteristic dimension of the object l , as described by equation (1): If Δ V is big enough, redox reactions can be carried out at the opposite sides of the particle, oxidation reactions at the anodic pole, simultaneously with reduction reactions at the cathodic pole. A large variety of applications using bipolar electrochemistry has been recently developed [29] , [30] , with a strong focus on material science [31] , [32] , [33] and analytical chemistry [29] . Bipolar electrochemistry has also been used directly or indirectly for the propulsion of objects. On one hand it is a straightforward approach for the synthesis of asymmetric microswimmers [17] , [34] and on the other hand it can induce a deposition/dissolution process, leading to the apparent motion of metal objects [35] . In the present contribution the key issue is to introduce bipolar electrochemistry as a concept for the site-selective generation of gas bubbles, which will in fine lead to the controlled locomotion of the polarized objects. In the present work we report on such use of electric fields for the polarization of conducting objects, which induces two spatially separated electrochemical reactions, involving directionally controlled gas bubble evolution that will trigger the motion of the object. We take advantage of the intrinsic asymmetric reactivity offered by this type of bipolar electrochemistry to propose a promising alternative mechanism that allows the propulsion of conducting objects in a controlled way. Electric field-induced linear motion Like many other redox reactions, water splitting can also be carried out at both extremities of a bipolar object. In an aqueous solution, the following reactions take place ( Fig. 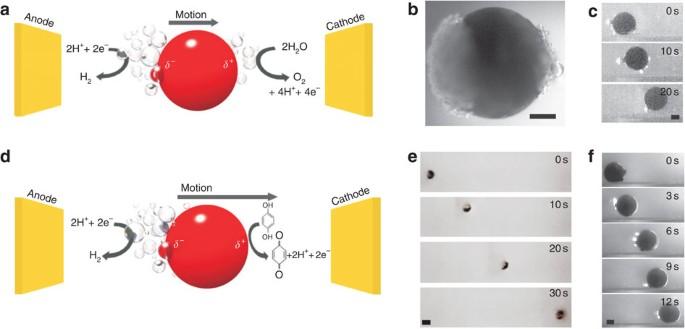Figure 1: Linear motion of spherical objects. (a–c) Competing bubble production. (a) Scheme of the water splitting by bipolar electrochemistry. (b) Optical micrograph of a stainless steel 1 mm spherical metal particle exposed to a 1.6 kV m−1electric field in aqueous 24 mM H2SO4. The left part of the bead is the cathodic pole where H2bubbles are produced and the right part is the anodic pole where O2bubbles are produced. Scale bar, 250 μm. (c) Translational motion generated with a 285-μm glassy carbon sphere in a PDMS microchannel exposed to a 5.3 kV m−1electric field in aqueous 7 mM H2SO4. Scale bar, 100 μm. (d–f) Quenching of O2bubble production. (d) Scheme of proton reduction and HQ oxidation. (e) Translational motion generated on a 1-mm stainless steel bead exposed to a 1.3 kV m−1electric field in 24 mM HCl and 48 mM HQ. Scale bar, 1 mm. (f) Translational motion generated with a 275-μm glassy carbon sphere in a PDMS microchannel with a 4.3 kV m−1electric field in an aqueous solution of 7 mM HCl and 14 mM HQ. Scale bar, 100 μm. 1a ): Figure 1: Linear motion of spherical objects. ( a–c ) Competing bubble production. ( a ) Scheme of the water splitting by bipolar electrochemistry. ( b ) Optical micrograph of a stainless steel 1 mm spherical metal particle exposed to a 1.6 kV m −1 electric field in aqueous 24 mM H 2 SO 4 . The left part of the bead is the cathodic pole where H 2 bubbles are produced and the right part is the anodic pole where O 2 bubbles are produced. Scale bar, 250 μm. ( c ) Translational motion generated with a 285-μm glassy carbon sphere in a PDMS microchannel exposed to a 5.3 kV m −1 electric field in aqueous 7 mM H 2 SO 4 . Scale bar, 100 μm. ( d–f ) Quenching of O 2 bubble production. ( d ) Scheme of proton reduction and HQ oxidation. ( e ) Translational motion generated on a 1-mm stainless steel bead exposed to a 1.3 kV m −1 electric field in 24 mM HCl and 48 mM HQ. Scale bar, 1 mm. ( f ) Translational motion generated with a 275-μm glassy carbon sphere in a PDMS microchannel with a 4.3 kV m −1 electric field in an aqueous solution of 7 mM HCl and 14 mM HQ. Scale bar, 100 μm. Full size image At the cathodic and anodic pole of the object, gas bubbles are produced that can be visualized as shown in Figure 1b on a 1-mm metallic bead located in a 1.6 kV m −1 electric field. To maintain electroneutrality at the bipolar electrode, the electron production and consumption must be equal at both sides. As a result, considering reactions 2 and 3, the produced hydrogen (H 2 ) volume (left side) is twice the produced oxygen (O 2 ) volume (right side). In analogy with chemically powered nanomotors [4] , [6] , [7] , this asymmetric bubble production is responsible for a directional motion. Figure 1c shows a conductive microswimmer that is propelled by using this mechanism. The 285-μm sized bead is moving towards the cathode in a polydimethylsiloxane (PDMS) microchannel at a speed of 20 μm s −1 , which corresponds to one body length every 14.2 s. As at this scale Brownian motion is negligible, this speed has been simply calculated by measuring the distance as a function of time. As the produced O 2 bubbles hinder this motion, one can increase the speed by suppressing this reaction, like illustrated in Figure 1d . The lower redox potential of the hydroquinone (HQ)/benzoquinone (BQ) redox couple, compared with the oxidation potential of water, makes it an ideal couple for suppressing the O 2 production. In an aqueous HQ solution, the following reactions happen at the cathodic and anodic poles of the bipolar object, respectively: In this case the bubble formation takes place only at the cathodic side of the object, leading to a higher speed. In the experiment that is reported in Supplementary Movie 1 and Figure 1e , a metal bead (diameter 1 mm) is propelled over a distance of 1.5 cm with a speed of 512 μm s −1 (about 1 body length every 2 s) by an electric field of 1.3 kV m −1 . According to equation (1), the potential difference Δ V that is generated between the two sides of the bead is 1.3 V, a value that is in agreement with the thermodynamic value corresponding to the combination of both reactions, if one takes into account that overpotentials are involved for both the reactions and that the reactions are not occurring under thermodynamic standard conditions. These coupled redox reactions can be used to move the object under various pH conditions, because the potential of proton reduction and HQ oxidation will shift by 60 mV per pH unit in the same direction, which means that the overall polarization, needed to drive the two reactions simultaneously, will remain the same. For micrometre-sized objects, as in the experiment reported in Supplementary Movie 2 and Figure 1f , a higher electric field is required to induce a Δ V of the same order of magnitude. An electric field of 4.3 kV m −1 was applied, which corresponds to a Δ V of 1.18 V across the 275-μm-sized glassy carbon bead. We used in this case, glassy carbon to illustrate that it is a quite general phenomenon that not only occurs on metal objects. On the basis of the data of Figure 1f , the bead velocity is 62 μm s −1 , or 1 body length every 4.4 s. Watching the imperfections on the bead surface in Supplementary Movie 2 , one can easily note that the bead is rolling inside the microchannel while moving. These imperfections are certainly also responsible, like surface roughness in general, for the bubble nucleation and release; however, no attempts were made to control this parameter, except that a surfactant has been added to the solution to decrease the size and the adherence of the bubbles to the surface. This leads to a more homogeneous release and thus also a more regular motion of the objects. It becomes also clear from the movie that the motion is due to the hydrodynamics produced by the local bubble release as a consequence of the bipolar reaction, and not due to other electrokinetic phenomena. In addition a control experiment carried out using an isolating glass bead did not lead to any movement. From this, one can conclude that under the present conditions, electroosmotic flow is not playing a significant role; however, it might become important when going to higher electric fields or for objects of smaller dimensions. The difference of measured velocity in the two experiments is mainly due to three parameters, that is, the difference in the generated Δ V values, the difference of hydrochloric (HCl) acid and HQ concentrations, which influences the reaction kinetics and thermodynamic parameters, and the different composition of the objects. This latter point is crucial, because different materials have different overpotentials/activation energies for carrying out a certain redox reaction. In particular it is more difficult to reduce protons on the carbon beads compared with the metal beads. Therefore, one can expect that in the latter case the local current that results in H 2 production will be higher compared with the one on carbon. This means that for the same external driving voltage more bubbles will be produced per time unit on the metal bead, leading in fine to more efficient propulsion and thus a higher speed. This shows that the speed of the objects can be controlled by using different experimental parameters. The concept has nevertheless some limits in terms of particle size. First of all when the objects become too small (typically in the micron or submicron range), viscosity effects become very important and therefore momentum-based propulsion is increasingly difficult. The friction that the particle has to overcome in order to move is amplified, due to the disadvantageous evolution of the surface to volume ratio. Second, the particles are more and more subjected to Brownian motion and therefore more force/energy has to be applied to fight against this. Finally, the external driving force, necessary in our experiment to generate a sufficient polarization, scales inversely with the particle diameter. This means that for moving smaller objects one needs larger fields, which is somewhat counterintuitive, because usually bigger objects need a bigger external driving force. As a direct consequence, very high external electric fields in the 1 MV m −1 range are necessary if one wants to trigger the water-splitting reaction on objects with a size in the submicrometre range. Electric field-induced rotational motion The described concept is not only efficient for inducing linear translation of objects but can also be adapted to generate rotational motion. We designed two kinds of bipolar electrochemical rotors, the first one rotating in a horizontal plane ( Fig. 2a ) and the second one in a vertical plane ( Fig. 4a ). 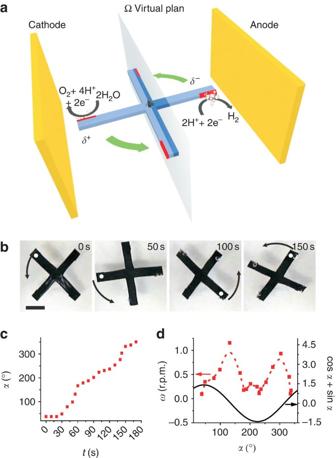Figure 2: Horizontal bipolar rotor. (a) Scheme of a horizontal rotor powered by bipolar electrochemistry-induced water splitting; red areas represent the conductive parts exposed to the solution, whereas the blue areas have been shielded with an insulating polymer. (b) Rotational motion of a horizontal bipolar rotor made out of a conducting polycarbonate sheet in an electric field of 0.5 kV m−1in 50 mM HCl. Scale bar, 0.5 cm. (c) Plot of the rotation angleαas a function of timet. (d) Plot of the experimental rotor speedω(red curve) compared with the theoretical variation of driving force (black curve) as a function of the rotation angleα. Figure 2: Horizontal bipolar rotor. ( a ) Scheme of a horizontal rotor powered by bipolar electrochemistry-induced water splitting; red areas represent the conductive parts exposed to the solution, whereas the blue areas have been shielded with an insulating polymer. ( b ) Rotational motion of a horizontal bipolar rotor made out of a conducting polycarbonate sheet in an electric field of 0.5 kV m −1 in 50 mM HCl. Scale bar, 0.5 cm. ( c ) Plot of the rotation angle α as a function of time t . ( d ) Plot of the experimental rotor speed ω (red curve) compared with the theoretical variation of driving force (black curve) as a function of the rotation angle α . Full size image Figure 4: Vertical rotor. 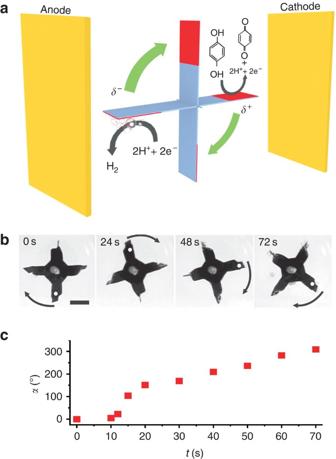Figure 4: Vertical rotor. (a) Scheme of a vertical rotor powered by the reduction of protons coupled to HQ oxidation. (b) Rotational motion of a vertical bipolar rotor, made out of a conductive polycarbonate sheet, in an electric field of 0.5 kV m−1in 50 mM HCl and 100 mM HQ. Scale bar, 0.5 cm. (c) Plot of rotation angleαas a function of timet. ( a ) Scheme of a vertical rotor powered by the reduction of protons coupled to HQ oxidation. ( b ) Rotational motion of a vertical bipolar rotor, made out of a conductive polycarbonate sheet, in an electric field of 0.5 kV m −1 in 50 mM HCl and 100 mM HQ. Scale bar, 0.5 cm. ( c ) Plot of rotation angle α as a function of time t . Full size image Supplementary Movie 3 and Figure 2b shows the rotation of a horizontal rotor powered by bipolar electrochemistry-induced water splitting. The rotor, a carbon-doped polycarbonate cross is supported by a thin glass needle axis, fixed at the bottom of the cell. To concentrate the bubble production on specific sites, the rotor surface has been shielded with an insulating polymer (blue parts in Fig. 2a ), except the extremities (red parts in Fig. 2a ). As in the case of the translational motion, the water-splitting reaction is induced at the extremities of the object by imposing an electric field of 0.5 kV m −1 , corresponding to a Δ V of 8.5 V. While rotating, the electroactive parts of the cross invert their polarization, when passing the virtual plane Ω parallel to the external electrodes and including the rotor axis. The conducting parts on the cross are positioned in such a way that an anticlockwise motion is generated. A rotational average speed of 1.9° s −1 has been calculated, which correspond to 0.32 r.p.m. However, this speed is not completely constant in time as can be seen in Figure 2c . 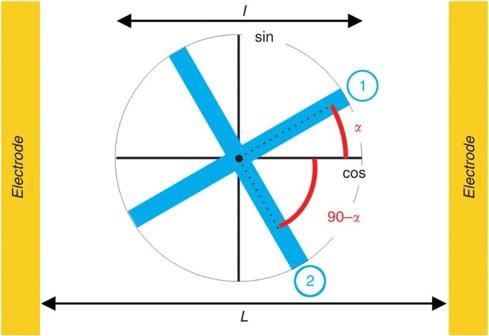This can be understood by considering the theoretical polarization of the object as a function of time. Figure 3: Theoretical rotor polarization. Scheme illustrating the variation of driving force for the whole object as a function of the angleαwith respect to the external electrodes.Lis the distance between the electrodes andlthe rotor diameter. Figure 3 illustrates that when the cross is exposed to the external electric field, the polarization voltage of the rotor arm 1 can be expressed as Δ V = E l cos α and the one of arm 2 as Δ V = E l sin α . Figure 3: Theoretical rotor polarization. Scheme illustrating the variation of driving force for the whole object as a function of the angle α with respect to the external electrodes. L is the distance between the electrodes and l the rotor diameter. Full size image Therefore, the overall polarization voltage, which is the driving force for propulsion, can be expressed as Δ V = E l (sin α +cos α ). This induces an acceleration of the rotor, and will lead to a maximum speed with a theoretical shift of 90° with respect to the maximum of the driving force. The experimentally obtained variation in speed is qualitatively in agreement with this theoretical function (see Fig. 2d ), and one observes in the beginning of the experiment indeed a good correlation between the theoretical maximum of the driving force, which appears at an angle of α =45°, and the maximum of experimental rotor speed which is located around 140°. The further velocity oscillations are slightly shifted with respect to the theoretically expected values, most likely because the size of the bubbles and the time when they detach from the blade is subject to random fluctuations. A control experiment with a completely insulated cross resulted in no rotation, demonstrating that this motion is exclusively due to bipolar electrochemistry. A vertical rotor can also be designed and is a very good option to enhance the rotational speed, as this configuration takes advantage of the buoyancy of the bubbles generated below the rotor blade. Actually, in general, when gas is released from the object, and while the resulting bubble is still attached to the object, the expansion of the gas bubble in the liquid exerts a force on the object, which pushes the latter one in the opposite direction [36] . In the particular case of the vertical rotor, the gas bubbles are sticking to the rotor blade and are located below the rotor blade because the rotor has been designed on purpose in that manner. This means that in addition to the above mentioned force, the buoyancy of the gas exerts a second type of force on the rotor blade ( Fig. 4a , left side), thus, leading in principle to a higher speed. However, if the bubbles adhere too strongly to the blade they will slow down the motion once they are dragged downwards (right side of the rotor). Therefore, one has to make sure that they will detach from the rotor when the blade is in the vertical position, essentially by the addition of small amounts of surfactant. The speed can be further optimized by suppressing again the O 2 evolution, occurring at the opposite blade, by adding HQ, because, again, generated O 2 bubbles might stick to the blade, and in this case, buoyancy slows down the rotation, because the forces are orientated in the wrong direction. A beneficial side-effect of using HQ is an increase in H 2 bubble production at the cathodic pole for the same external electric field, because a lower Δ V is required for the combination of these two redox reactions. This leads to a higher velocity. Supplementary Movie 4 and Figure 4b illustrates the motion of a vertical rotor exposed to a Δ V of 8.5 V. The motion seems to be slightly more homogeneous ( Fig. 4c ) than in the horizontal configuration and the extrapolated average rotational speed is 4.2° s −1 (0.70 r.p.m. ), more than two times higher compared with the previous speed. Although one would expect in this case as well a sigmoid variation of the angular speed, it is levelled out by the buoyancy effect, specific to this setup. Changing different parameters such as the solution composition and the rotor design, the efficiencies can be optimized and one can imagine that this kind of rotors could be used for producing additional mechanical energy in a setup where electric fields are used anyway, such as in electrolysis reactors. From the above-presented results it can be concluded that bipolar electrochemistry can be used for inducing motion of objects. Control experiments showed that this motion is not due to one of the usual propulsion mechanisms such as self-electrophoresis, diffusiophoresis or electroosmotic flow. It is therefore a new concept for chemical locomotion, based on the polarization of a conducting object, which triggers chemical reactions that imply gas bubble evolution, inducing in fine a linear or rotational motion of the object. The induced motion is not completely regular, on one hand due to the somewhat random detachment of the bubbles from the object and on the other hand due to intrinsic variations in polarization intensity as for the rotors. In the latter case an increase of the number of rotor arms can smooth this kind of variations. The illustrated approach is an original alternative to classical propelling mechanisms. Compared with intrinsically asymmetric swimmers [4] , [5] , [6] , [7] , in this case, the electric field induces the asymmetric reactivity. It is possible to switch from linear to rotational motion by changing the design of the setup. The approach is very versatile because the moving objects can be made out of various kinds of conductive materials with different shapes and sizes. Here we have demonstrated in a series of proof-of-principle experiments that it is possible to induce motion at the macroscopic and microscopic scale; however, the mechanism has a lower experimental limit in the micrometre range due to the inherent restrictions in applied electric field, which scales inversely with the size of the object. The concept could be in principle extended to moving particles in the x – y plane or even in three dimensions when a multi-electrode setup is used. One can imagine various applications of this mechanism, ranging from carrying cargo in microfluidic chips to the transformation of electrical into mechanical energy, for example, in electrolysis cells. Preparation of solutions All chemicals were used as received; solutions were prepared using Milli-Q water (resistivity=18 MΩ cm). For the motion experiments, a few drops of surfactant (Gojo NXT) were added to the solutions to decrease the bubble size and their adherence to the surface of the objects. The glassy carbon beads (spherical powder 200–400 μm type 1) were supplied by Alfa Aesar. 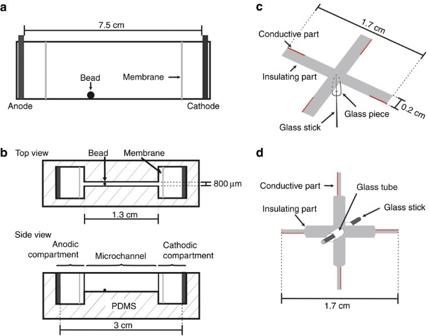Figure 5: Electrochemical cell and rotor description. (a) Side view of the setup used for the propulsion of 1 mm stainless steel beads. (b) Cell used for the propulsion of micrometre-sized glassy carbon beads. (c) Horizontal rotor scheme. (d) Vertical rotor scheme. Electrochemical cells The homemade cells we used are presented in Figure 5a and 5b . They were made out of PDMS or glass. In the latter case the different parts were sealed with silicon rubber. Cation-exchange membranes were supplied by the NCBE. To observe the moving objects a Zeiss Axiovert 25 microscope has been used, together with a Zeiss AxioCam MRm or a Sony Cyber-shot camera. The linear motion has been monitored in the transmission mode under the microscope. Figure 5: Electrochemical cell and rotor description. ( a ) Side view of the setup used for the propulsion of 1 mm stainless steel beads. ( b ) Cell used for the propulsion of micrometre-sized glassy carbon beads. ( c ) Horizontal rotor scheme. ( d ) Vertical rotor scheme. Full size image Linear motion generated on a 1-mm bead For the linear motion of the 1-mm stainless steel bead, the used cell is presented in Figure 5a . The electric field was imposed by applying a 100-V bias between the two platinum electrodes. The electrodes were separated by cation-exchange membranes. The cell was filled with a 24-mM HCl and a 48-mM HQ solution in water, and the bead is placed between the two membranes. The motion was recorded from the top using a digital camera. For the control experiment a glass bead with a diameter of 2.3 mm has been exposed to voltages of up to 130 V in the cell presented in Figure 5a . Linear motion generated on micrometre-sized beads The setup used for the linear motion of the micrometre-sized bead is presented in Figure 5b . The 800-μm-wide PDMS microchannel with an open top side was designed by using a PDMS kit. Cation-exchange membranes were also included to separate the microchannel from the electrode compartments. Electrodes were platinum sheets. The cell was filled with 24 mM H 2 SO 4 or 7 mM HCl and 14 mM HQ aqueous solutions. The glassy carbon bead was placed in the microchannel and the motion was recorded from the bottom using the CCD camera mounted on an optical microscope. Rotation of a horizontal bipolar rotor The horizontal rotor scheme is represented in Figure 5c . The rotor is made by cutting a polycarbonate sheet doped with carbon particles (Bayer). Some parts of the surface were insulated by coating with a varnish layer. Glass parts were made by melting glass capillaries and adjusting them into the desired shapes. In the centre of the cross, a small glass cup was fixed and positioned on top of a very thin glass stick. The cell described in Figure 5a was used for the rotation experiments with a 37-V bias. The motion was recorded from the top using a digital camera. How to cite this article: Loget, G. et al . Electric field-induced chemical locomotion of conducting objects. Nat. Commun. 2:535 doi: 10.1038/ncomms1550 (2011).